Spatially resolved one-dimensional boundary states in graphene–hexagonal boron nitride planar heterostructures Two-dimensional interfaces between crystalline materials have been shown to generate unusual interfacial electronic states in complex oxides. Recently, a one-dimensional interface has been realized in hexagonal boron nitride and graphene planar heterostructures, where a polar-on-nonpolar one-dimensional boundary is expected to possess peculiar electronic states associated with edge states of graphene and the polarity of boron nitride. Here we present a combined scanning tunnelling microscopy and first-principles theory study of the graphene–boron nitride boundary to provide a first glimpse into the spatial and energetic distributions of the one-dimensional boundary states down to atomic resolution. The revealed boundary states are about 0.6 eV below or above the Fermi level depending on the termination of the boron nitride at the boundary, and are extended along but localized at the boundary. These results suggest that unconventional physical effects similar to those observed at two-dimensional interfaces can also exist in lower dimensions. The ability to control the interfacial properties at the boundary between different materials has formed one of the foundations of modern condensed matter physics and device technology [1] , [2] , [3] , [4] , [5] . With the advent of graphene and other two-dimensional (2D) crystals, one-dimensional (1D) equivalents of conventional interfaces are envisioned: linear boundaries separating dissimilar materials joint in a single 2D atomic sheet. Graphene and hexagonal boron nitride (hBN) offer a prototypical system to build such a 2D heterostructure [6] , [7] , [8] , [9] , [10] , [11] . They are isostructural, nearly lattice-matched and isoelectronic, yet their different band structures and the polar-on-nonpolar boundary promise interesting properties arising from their 2D heterostructures [12] , [13] , [14] , just as for interfaces in the three-dimensional (3D) counterparts [1] , [2] , [3] , [4] , [5] . Indeed, the graphene–hBN zigzag boundary is predicted to possess peculiar boundary states [12] , [13] , [14] . Half-metallicity has been reported at this boundary based on theoretical calculations [15] , [16] , [17] , [18] , [19] , although zigzag graphene nanoribbons have insulating edge states [13] , [20] , [21] , [22] , [23] . Despite the enormous interest in graphene–hBN heterostructures, the theoretically expected boundary states have not yet been validated experimentally. Some early attempts to address the boundary states have been focused on the connections between graphene and a metallic supporting substrate. For example, when a graphene island is bonded to the edges of a Pt(111) step, a boundary state is shown to be associated with specific sublattices of the graphene structure [24] . On the other hand, graphene nano-islands grown on Ir(111) do not show boundary states as the graphene edges are hybridized with the substrate, and the edge states at Ir(111) are quenched by the strong interaction between the metal and the graphene [25] . Moreover, in a 3D polar-on-nonpolar heterostructure of such as Ge–GaAs or LaAlO 3 –SrTiO 3 , the polar discontinuity introduces an electric field, which could create an unsustainable electrostatic potential at the interface (termed as the ‘polar catastrophe’ [26] ), leading to electronic or atomic reconstructions [3] , [5] , [26] , [27] and even preventing an atomically sharp boundary in the latter case [5] , [27] . It is unclear whether such a polar catastrophe would occur in a 2D polar-on-nonpolar heterostructure of graphene–hBN. Here we combine scanning tunnelling microscopy (STM) and first-principles theory methods to study the spatial and energetic distributions of the electronic boundary states in the graphene–hBN in-plane heterostructures. The interfaces studied here are crystallographically coherent with sharp transitions from graphene zigzag edges to B (or N)-terminated monolayer hBN on a Cu foil substrate [6] . The boundary states are revealed down to the atomic level with energy levels about 0.6 eV below and above the Fermi level, respectively, for the B- and N-terminated boundaries. The boundary states are shown to be extended along the boundary, and exponentially decay into the bulk of graphene and hBN with decay lengths in a range of 0.24–0.51 nm. The boundary states come from the mixing of π orbitals of C, B and N at each edge, with the occupied bonding states ( π CB ) at B-terminated edges and the unoccupied anti-bonding states ( π * CN ) at N-terminated edges. The effect of the electric field induced by the polarity discontinuity at the interface is discussed, which can be effectively screened out by the charge carriers from graphene and Cu substrate. STM topography of graphene–hBN heterostructures An in-plane, single-atomic layer graphene–hBN heterostructure grown on a Cu foil [6] is used to experimentally investigate the boundary states in this work owing to the weak substrate interaction [28] and a sharp boundary at the atomic scale [6] . 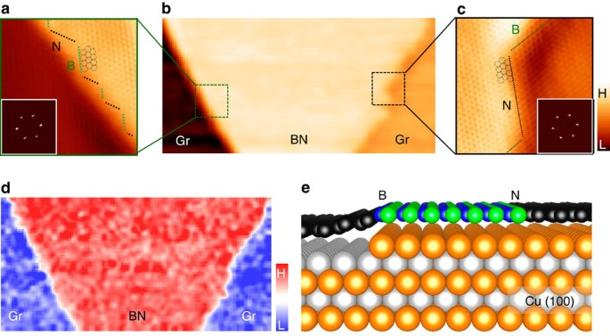Figure 1: STM topography of a planar graphene–hBN–graphene heterostructure. (a–c) STM images, with large-scale image inbshowing two adjacent boundaries (50 × 25 nm2, 0.5 V, 200 pA), andaandcshowing atomically resolved images near each boundary (6 × 6 nm2). The edge terminations of hBN are marked with dotted lines. Insets: fast Fourier transform from the images. (d) Simultaneously obtained dI/dVmap with image inb(AC modulation 500 Hz, 50 mV). (e) Schematic illustration of two boundaries on Cu(100) substrate projected along <011>direction. The height difference of the two junctions is due to an underlying Cu(100) step (Δh=1.8 Å). ‘B’ and ‘N’ indicate the hBN region termination, determined by STS in conjunction with first-principles calculations. Gr and BN represent graphene and hBN regions for simplicity. Figure 1b shows an STM image of two adjacent graphene–hBN junctions formed by an hBN region between two graphene regions, with magnified images of the respective boundaries shown in Fig. 1a and Fig. 1c . The zigzag boundary orientations are indicated in Fig. 1a,c . The image contrast in Fig. 1a is dominated by a substrate step, which appears to be close to an armchair orientation. However, superimposing the schematic atomic lattice on the image and comparing with d I /d V map (details shown in Supplementary Fig. 1 ) reveal that the structures of the boundary are actually zigzag. The simultaneously acquired scanning tunnelling spectroscopy (STS) map ( Fig. 1d ) shows distinctively different contrasts between graphene (blue) and hBN (red) regions. Our assignments of graphene and hBN regions are based on STS measured across the boundaries ( Supplementary Figs 2 and 3 ), where graphene and hBN show distinctively different characteristics with graphene showing a dip at Dirac point of -0.35 V and the hBN showing a large band gap of ~4 eV (refs 6 , 29 , 30 , 31 , 32 ). The boundary on the right side ( Fig. 1c ) shows a small height difference (~ 0.7 Å) originating from the difference in the electronic density of states between the graphene and hBN, and the left boundary ( Fig. 1a ) has a height difference of 2.5 Å that consists of a substrate step (1.8 Å) on Cu(100), the predominant surface orientation of the Cu foil substrate [6] , [29] ( Supplementary Fig. 4 ). Figure 1e depicts a schematic of these two boundaries on the substrate. Figure 1: STM topography of a planar graphene–hBN–graphene heterostructure. ( a – c ) STM images, with large-scale image in b showing two adjacent boundaries (50 × 25 nm 2 , 0.5 V, 200 pA), and a and c showing atomically resolved images near each boundary (6 × 6 nm 2 ). The edge terminations of hBN are marked with dotted lines. Insets: fast Fourier transform from the images. ( d ) Simultaneously obtained d I /d V map with image in b (AC modulation 500 Hz, 50 mV). ( e ) Schematic illustration of two boundaries on Cu(100) substrate projected along <011>direction. The height difference of the two junctions is due to an underlying Cu(100) step (Δ h =1.8 Å). ‘B’ and ‘N’ indicate the hBN region termination, determined by STS in conjunction with first-principles calculations. Gr and BN represent graphene and hBN regions for simplicity. Full size image The boundary structures are further confirmed by simultaneously acquired atomic-resolution STM images and STS maps. As shown in Supplementary Fig. 2 , all the graphene–hBN boundaries are found to contain some segments oriented 120° away from the primary edge direction, which have different terminations than the primary edges, considering the lattice symmetry of hBN and that a zigzag interface is more energetically favourable (about 1.37 eV per edge carbon atom) than a Klein-type interface [33] for this graphene–hBN heterostructure on a Cu substrate. By comparing measured boundary states with theoretical analysis (discussed later), we identify boundary terminations as indicated in Fig. 1a,c . Energetic distributions of boundary states We now examine the electronic properties of both B- and N-terminated graphene–hBN boundaries by measuring the differential conductance d I /d V , which is proportional to the local electronic density of states (LDOS) distribution, especially at low bias voltages. 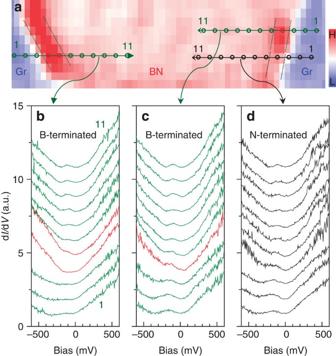Figure 2: Electronic boundary states measured by STS. (a) dI/dVconductance map (45 × 12.5 nm2) of the Gr–hBN–Gr regions measured at -0.6 V to the sample. The boundary states (between green dotted lines) are noticeable as intense red colour. Circles on arrowed lines mark positions of STS from graphene to the hBN, where green lines go across the B-terminated regions and black lines across the N-terminated region. (b–d) dI/dVcurves acquired along three lines marked ina. The red curves correspond to those acquired between green dotted lines ina. Spectroscopy data are offset for clarity. Figure 2a shows the d I /d V map at a bias voltage of −0.6 V for the two boundaries displayed in Fig. 1b . The electronic states can be seen at both boundaries as intense red-coloured regions. Enhanced electronic states are observed only at the B-terminated boundaries (indicated by green dotted lines), not at the N-terminated boundary (indicated by black dotted lines) at this bias voltage. The measured d I /d V curves in Fig. 2b–d show LDOS variations along three different lines going from graphene to hBN as indicated in Fig. 2a . Remarkably, the d I /d V curves at the B-terminated boundaries (red curves) display enhanced LDOS at around −0.6 V that corresponds to the intense red-coloured region in the d I /d V map ( Fig. 2a ). On the other hand, the N-terminated boundary ( Fig. 2d ) does not show an increase in LDOS at −0.6 V; instead, it shows highly localized electronic states at positive bias as explained below. Figure 2: Electronic boundary states measured by STS. ( a ) d I /d V conductance map (45 × 12.5 nm 2 ) of the Gr–hBN–Gr regions measured at -0.6 V to the sample. The boundary states (between green dotted lines) are noticeable as intense red colour. Circles on arrowed lines mark positions of STS from graphene to the hBN, where green lines go across the B-terminated regions and black lines across the N-terminated region. ( b – d ) d I /d V curves acquired along three lines marked in a . The red curves correspond to those acquired between green dotted lines in a . Spectroscopy data are offset for clarity. Full size image Spatial distributions of boundary states The spatial confinement of boundary states can be visualized clearly by plotting the measured d I /d V intensity contours at a constant bias voltage. 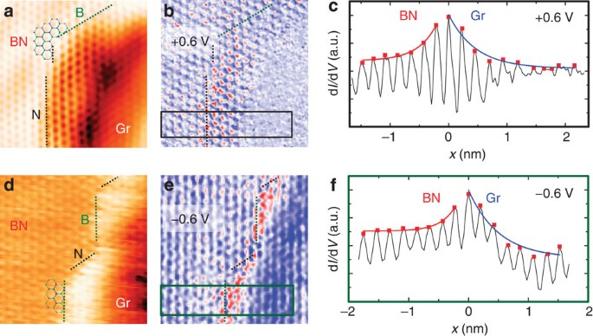Figure 3: Spatial distributions of boundary states. (a,d) Atomically resolved topography image of planar junction showing the seamless connections between graphene (right) and hBN (left) regions. (b,e) Simultaneously obtained dI/dVconductance map with the images (a,d) displaying distinct boundary states in red (with the same colour scheme as shown inFig. 2a) at different bias voltages with the same set point (200 pA). Image sizes:aandb, 4.2 × 4.2 nm2;dande, 4 × 4 nm2. Hexagonal lattice of hBN is overlaid on topography. Green and black dotted lines indicate B- and N-terminated boundaries, respectively. (c,f) Averaged line profiles across the boundary regions (marked with boxes inbande) showing exponential decay of the interfacial state into the both graphene and hBN regions. Red and blue lines are exponential fitting curves. Figure 3b shows the atomically resolved spatial distributions of measured d I /d V across a graphene–hBN boundary, acquired simultaneously with the STM image ( Fig. 3a ) at 0.6 V. At this bias, the LDOS enhancement appears only at N-terminated edges, and is confined within a few atomic lattices near the boundary. Moreover, the d I /d V intensity at constant bias decays exponentially from the boundary into the graphene and hBN regions ( Fig. 3c ). We find that the boundary state decays slightly faster in hBN than in graphene, with a larger decay length on the graphene side (0.47±0.08 nm) than the hBN side (0.32±0.05 nm). In contrast, the B-terminated boundary states become more pronounced at −0.6 V as shown in Fig. 3d–f with decay lengths of 0.51±0.17 and 0.24±0.05 nm on the graphene and the hBN side, respectively. Figure 3: Spatial distributions of boundary states. ( a , d ) Atomically resolved topography image of planar junction showing the seamless connections between graphene (right) and hBN (left) regions. ( b , e ) Simultaneously obtained d I /d V conductance map with the images ( a , d ) displaying distinct boundary states in red (with the same colour scheme as shown in Fig. 2a ) at different bias voltages with the same set point (200 pA). Image sizes: a and b , 4.2 × 4.2 nm 2 ; d and e , 4 × 4 nm 2 . Hexagonal lattice of hBN is overlaid on topography. Green and black dotted lines indicate B- and N-terminated boundaries, respectively. ( c , f ) Averaged line profiles across the boundary regions (marked with boxes in b and e ) showing exponential decay of the interfacial state into the both graphene and hBN regions. Red and blue lines are exponential fitting curves. Full size image These boundary states are reproducibly observed in an energy range of 0.45–0.78 eV below the Fermi level for the B-terminated boundaries and 0.60–0.90 eV above the Fermi level for the N-terminated boundaries (see Supplementary Figs 2,5,6 for more details), confirming that the appearance of these states are not experimental artefacts but an intrinsic boundary property. Moreover, all the boundary states are localized at and extended along the boundary, although the electronic states at B- and N-terminated boundaries have clearly different energy levels. First-principles calculations of boundary states We now compare the experimental observations with first-principles density functional theory (DFT) calculations (see Methods for the details). As illustrated in Fig. 4a , we consider a supercell in which an hBN ribbon of 7 zigzag rows joint by a 12-row graphene ribbon, on a 5-layer Cu slab, oriented (100) with a 0° rotation angle. In view of the experimentally identified superstructure (six graphene or hBN unit cells match to five Cu(100) surface lattice unit cells in the direction perpendicular to the boundary [6] ), graphene–hBN supercell is not unique. We consider a flat graphene–hBN on Cu(100) while excluding local lattice distortions that vary with supercell configurations. We project the density of states on each hBN or graphene zigzag row in the unit cell (see Supplementary Fig. 7 ). To facilitate the comparison of the calculated LDOS with the measured d I /d V , we plot the LDOS contour within a small energy region (from −0.8 eV to 0.4 eV) near the Fermi level in Fig. 4b,c for the B- and N-terminated boundaries, respectively, with the contribution from Cu excluded for clarity. For the B-terminated boundary ( Fig. 4a ), the boundary states are located about 0.6 eV below the Fermi level and localized within only a few rows (row-to-row distance is 2.165 Å, given a 1.44-Å C–C or B–N length) of the interface. The spatial distribution of LDOS extends into the graphene region more deeply than into the hBN region, with the decay length in graphene 3.1 Å and in hBN 2.0 Å, respectively. The highest intensity of LDOS appears at the C site for both B- and N-terminated boundary states, consistent with the measured d I /d V ( Fig. 3c,f ). Both the calculated energy position of the B-terminated boundary state and its decay length are in good agreement with the STS measurement. 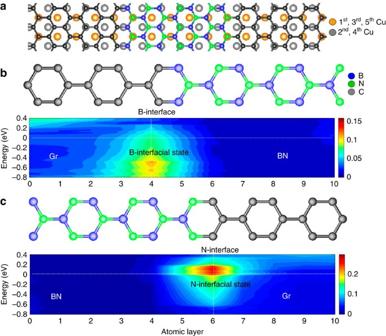Figure 4: Calculated boundary states of the planar graphene–hBN–graphene heterostructure on a Cu(100) substrate. (a) Schematic of the heterostructure (top view). Seven hBN zigzag rows are laterally sandwiched by 12 graphene rows. Five Cu layers are considered as the substrate. B atoms are specified in blue, N atoms in green and carbon atoms in black. (b) Contour map related to the B-terminated state made up of LDOS projected onto 11 zigzag rows (5 graphene and 6 hBN rows) across the B-terminated boundary. B-terminated states are located around 0.6 eV below the Fermi level. (c) Contour map related to the N-terminated state across the N-terminated boundary. The boundary states are located around 0.1 eV above the Fermi level. Figure 4: Calculated boundary states of the planar graphene–hBN–graphene heterostructure on a Cu(100) substrate. ( a ) Schematic of the heterostructure (top view). Seven hBN zigzag rows are laterally sandwiched by 12 graphene rows. Five Cu layers are considered as the substrate. B atoms are specified in blue, N atoms in green and carbon atoms in black. ( b ) Contour map related to the B-terminated state made up of LDOS projected onto 11 zigzag rows (5 graphene and 6 hBN rows) across the B-terminated boundary. B-terminated states are located around 0.6 eV below the Fermi level. ( c ) Contour map related to the N-terminated state across the N-terminated boundary. The boundary states are located around 0.1 eV above the Fermi level. Full size image The calculations employing the DFT exchange and correlation (XC) functional of the local density approximation (LDA) also yield highly localized states at the N-terminated boundary located around 0.1 eV above the Fermi level ( Fig. 4c ), lower than that measured by STS mapping. As LDA calculations usually underestimate the band gaps and especially the energies of unoccupied states, we further performed Heyd−Scuseria−Ernzerhof (HSE) hybrid functional calculations [34] on a small supercell (see Methods for details) to account for the discrepancy in the N-terminated boundary state level. It is found that the energy level of B-terminated states remain unchanged from the LDA result on the same supercell, but the N-terminated states move up to~0.6 eV above the Fermi level (see Supplementary Fig. 8 ); and the shift accounts for the difference in the N-terminated boundary states between the experiment and the LDA results in Fig. 4c . Although the interactions with the Cu substrate are very weak [28] , we find that there are still hybridizations between the d -orbitals of Cu and the π -orbitals of graphene and hBN near the B-terminated boundary (see Supplementary Fig. 9 ). However, no appreciable interaction is seen between N-terminated states and Cu states. These dissimilar interactions arise from the different electronegativities of B and N. As a comparison, we have compared the calculated LDOS with and without a Cu substrate ( Supplementary Fig. 10 ) and found that the N-terminated boundary states remain largely unchanged, but the B-terminated states are modified by the Cu substrate due to the hybridization with Cu substrate. In comparison, we carried out DFT calculations on an in-plane graphene–hBN junction on Cu(111). As shown in Supplementary Fig. 11 , the calculated results for both B- and N-terminated boundaries are essentially the same as those on Cu(100), confirming that crystallographic orientation of Cu has little effect on the boundary states. We now clarify the nature of the observed boundary states on the basis of the combined experimental and theoretical study. When two semi-infinite sheets of graphene and hBN form a zigzag heterojunction on a Cu substrate, the mixing of π -orbitals of C, B and N at each edge gives rise to four sets of bands that correspond to the bonding and anti-bonding states between C–N and C–B ( Supplementary Fig. 12 ). Although the boundary states are spin polarized in the free-standing case [13] as are the edge states of free-standing zigzag hBN nanoribbons [35] , calculations by us and others [36] indicate that the boundary magnetism disappears upon adsorption onto a Cu substrate. The relevant bands, close to the Fermi level, are the occupied bonding states ( π CB ) at B-terminated edges and the unoccupied anti-bonding states ( π * CN ) at N-terminated edges, both localized at the interface. The localized states lay ~0.6 eV below and above the Fermi level, respectively ( Fig. 3 ). In addition, different electronegativities of B and N make the hBN strip the 2D equivalent to a polar slab. We calculated that a free-standing eight-row hBN strip experiences a polar field of ~0.11 eV Å −1 , which is reduced to about 0.06 eV Å −1 by screening when joint with graphene. The Cu substrate brings about an additional screening, as corroborated in our calculations. In a 3D polar-on-nonpolar heterostructure, 2D charge sheets create a constant overall electric field and the electrostatic potential would diverge with increasing thickness, leading to a ‘polar catastrophe’ [26] . The polar catastrophe can be averted by charge reconstruction [26] or atom rearrangement [5] . For (100) or (111) Ge–GaAs interfaces, which are the higher-dimensional analogies of the zigzag graphene–hBN boundaries, atom rearrangement prevents an atomically sharp interface [5] , [27] . In a 2D polar-on-nonpolar heterostructure, the electric field induced by the polar discontinuity at the boundary is inversely proportional to the distance, and the electrostatic potential would also diverge although not as fast as in 3D. Furthermore, the charge carriers from graphene and Cu substrate can effectively screen out the polar field. As such, the polarity discontinuity in 2D may not be as catastrophic. Nevertheless, planar graphene–hBN heterostructures provide an excellent platform for exploring novel physics in a 1D system—the interface in 2D space. Sample preparation and STM/STS experiments The graphene–hBN planar junction on Cu foil sample was prepared using the 2D heteroepitaxial growth technique [6] . Moreover, (100) has been found to be the predominant Cu surface orientation as confirmed by low-energy electron microscopy and low-energy electron diffraction [6] and X-ray diffraction and electron backscatter diffraction ( Supplementary Fig. 4 ). STM/STS were performed using a variable-temperature STM (Omicron) with Nanonis (SPECS) controller and an electrochemically etched tungsten tip. All measurements were carried out in ultra-high vacuum (<3 × 10 –10 Torr) at room temperature. We annealed the sample at 430 °C for 48 h for cleaning. We used constant current mode for topography images and a lock-in technique for differential conductance measurement with 500 Hz, 40–100 mV AC modulations. All STM images and spectroscopy data were analysed and processed with WSxM software. First-principles calculations First-principles calculations, based on DFT, were performed using the Vienna Ab initio Simulation Package. The projector-augmented wave method was used to mimic the ionic cores, while the LDA considering the Ceperly–Alder–Perdew and Zunger (CA-PZ) functional was employed for the XC functional. In addition, an HSE-screened hybrid XC functional [34] was used to more properly determine the energies of interface states. The overall fraction of Fock exchange and the length scale ω −1 for exchange screening are adopted as the HSE12s (ref. 37 ) form of a =0.425 and ω =0.408 Å –1 . Atomic positions, as well as lattice parameters, were optimized using a conjugate gradient algorithm. The ionic and electronic relaxations were performed by applying a convergence criterion of 5 × 10 −2 eV Å −1 per ion and 10 −4 eV per electronic step, respectively. The rectangular graphene–BN hybrid structure, 43.3 × 2.5 Å, is used for the LDOS calculations, and a vacuum of 16 Å between the hybrids is considered. Also, 1 × 10 × 1 Monkhorst–Pack meshes were used to perform the integration over the Brillouin zone. How to cite this article: Park, J. et al. Spatially resolved one-dimensional boundary states in graphene–hexagonal boron nitride planar heterostructures. Nat. Commun. 5:5403 doi: 10.1038/ncomms6403 (2014).